Understanding water’s anomalies with locally favoured structures Water is a complex liquid that displays a surprising array of unusual properties, the most famous being the density maximum at about 4 °C. The origin of these anomalies is still a matter of debate, and so far a quantitative description of water’s phase behaviour starting from the molecular arrangements is still missing. Here we report a study of the microscopic structural features of water as obtained from computer simulations. We identify locally favoured structures having a high degree of translational order in the second shell, and a two-state model is used to describe the behaviour of liquid water over a wide region of the phase diagram. Furthermore, we show that locally favoured structures not only have translational order in the second shell but also contain five-membered rings of hydrogen-bonded molecules. This suggests their mixed character: the former helps crystallization, whereas the latter causes frustration against crystallization. The anomalous thermodynamic and kinetic behaviour of water is known to play a fundamental role not only in many physical and chemical processes in materials science but also in biological, geological and terrestrial processes in nature [1] , [2] , [3] , [4] . For this reason, a lot of effort has been devoted to rationalizing water’s anomalous behaviour in a coherent and simple physical picture, but no consensus has yet emerged. One of the breakthroughs in this endeavour was the discovery of water’s polyamorphism, that is, the existence of amorphous coexisting phases in the supercooled region of the phase diagram. Distinct states have indeed been found in glassy water, called low-density, high-density and very high-density [5] amorphous ices, which can interconvert with each other by the application of pressure. Whether the transition between the amorphous ices has an equilibrium counterpart, with a first-order phase transition line above the glass transition temperature that terminates at a critical point (liquid–liquid critical point; LLCP), has become a matter of much controversy [6] , [7] , [8] , [9] , [10] , [11] , [12] , [13] , [14] . A major source of difficulty lies in the fact that most modern theories of water concentrate on the supercooled region of the phase diagram, which is difficult to access by experiments due to the rapid crystallization of water below its melting line [4] , [15] . Similar difficulties emerge also in simulations, where the lack of crystallization is sometimes hindered by the limited system sizes and timescales accessible [14] . From a pragmatic point of view, the existence of the homogenous crystallization line, below which the relaxation time of the liquid becomes shorter than the homogenous crystallization time, implies that, at the best of today’s knowledge, such supercooled liquid states will never be reached at bulk conditions, as already is found in simulations of coarse-grained water models [12] , [16] , [17] . Efforts to overcome this difficulty include either strong spatial confinement [18] or mixing an anti-freezing component [19] , [20] . Water anomalies are not located only in the supercooled regime (for example, the density maximum at 4 °C), and are not necessarily due to an underlying critical phenomena. A fundamental role is played by hydrogen bonds, as shown by modified Van der Waals theories that take into account states with optimal hydrogen bonding [21] , [22] . One way to understand water’s polyamorphic behaviour is to introduce the concept of locally favoured structures [23] , [24] , [25] , [26] , which are defined as particular long-lived molecular arrangements that correspond to some local minima of the free energy. In this view, water’s polyamorphism comes from the competition between two different types of molecular arrangements [3] : one in which the different tetrahedral units form open structures, and the other with a smaller specific volume due to a high degree of interpenetration. The presence of two amorphous fluid phases has indeed been observed in computer simulations of some models of water, where the freezing transition can be avoided [9] , [10] , [27] . The structuring of the fluid phase before crystallization has recently emerged as an important feature of supercooled liquids [25] , [28] , [29] . The idea that fluids are increasingly structured as they are supercooled was found to be very fruitful for a wide variety of systems [25] , [26] , including water [16] , [29] . According to this view, the structure of water is not just a random collection of states compatible with the overall hydrogen-bonding pattern, but special structural patterns emerge as the fluid is supercooled. In this work, we will try to connect directly the structuring of the fluid with the anomalous phase behaviour of water. The simplest model of water’s structure is then to assume the existence of two separate microscopic states. Many physical quantities exhibit behaviours suggestive of two states in liquid water, such as infrared and Raman spectra [1] , and the presence of an isosbectic point in Raman spectra has been regarded as a clear indication supporting a mixture model since its finding by Walrafen [30] . Some evidence for the inhomogenous structure of water was also reported in experimental studies of X-ray absorption spectroscopy, X-ray emission spectroscopy and X-ray small angle scattering [31] , [32] , but these results are highly debated [33] , [34] , especially since the majority component at room temperature was proposed to be associated with the break-up of the tetrahedral structure. Recently, evidence for two distinct local structures was found in the vibrational dynamics and relaxation processes in supercooled bulk water [35] . Despite these pieces of evidence supporting a two-state picture, the lack of a clear connection between these experimental observables and the amount of locally favoured structures has made it difficult to estimate the fractions of the two states in a convincing manner. From a phenomenological standpoint, two-state models have been extremely successful in describing the anomalies of water using a restricted number of fitting parameters [23] , [24] , [25] , [26] , [36] , and recent simulations by Cuthbertson and Poole [37] have opened the way for a quantitative assessment of these models from microscopic information, but only for state points around the Widom line, that is, at temperatures not accessible to experiments and far from the anomalies. For the same water model, the validity of a two-state model with excess free enthalpy (see equation (1)) has been recently assessed [38] . The essential difficulty in defining locally favoured states is finding a structural order parameter that directly correlates with water’s anomalies. Several attempts have been made, each differing in the microscopic definition of the states involved. Examples include states based on ice polymorphs [39] , tetrahedral order [32] , [40] , [41] or relative distance between neighbours [37] , [42] , [43] , [44] , [45] . To overcome this difficulty, we introduce a new structural order parameter that quantifies the degree of translational order in the second shell together with the information on intermolecular hydrogen bonding. We show that, for two of the most reliable computer models, water anomalies can be explained by the increase of translational ordering of the second shell with supercooling. We further identify the structural characteristics of the locally favoured structures of water and their link to the unusually large degree of supercooling of the liquid phase. Simulations We conducted molecular dynamics simulations of the TIP4P/2005 model of water, one of the best models of the liquid state [46] . Simulations were run for many state points covering a large area of the liquid state, with temperatures ranging from T =200 to 350 K, and pressures ranging from P =−1 to 3 kbar. To identify hydrogen bonds, we adopted the definition found in ref. 47 and which is widely used in simulations of liquid water, as mentioned above. Temperature is always expressed in K, pressure in bar, distance in nm, density ρ in g cm −3 and isothermal compressibility κ T in bar −1 . To show that our results are not limited to the TIP4P/2005 model potential, we also run simulations of the TIP5P potential (except for one section, all results in the manuscript are presented for the TIP4P/2005 potential). For more details on the simulation methods, refer to the Methods section. Relevant structural order parameter To identify locally favoured structures, we focus on a particular feature that characterizes the structure of supercooled liquid water, that is, the ordering of the second shell of nearest neighbours. To illustrate this point we plot in Fig. 1a the probability distribution for the distance between the first and second shell ( d f–s ) for different temperatures, from well above to well below melting. For each oxygen atom, the distance between the two shells is defined as the radial distance between the fifth and fourth nearest neighbours. The figure shows that at high temperatures, the distribution of d f–s is an exponentially decreasing function, which is the expected distribution for a fully disordered structure. As the temperature is lowered below melting, the liquid starts structuring and develops a finite separation between the first and second shells, approaching the distribution found in the solid phase, the hexagonal ice ( I h in the figure). The figure shows that supercooled water is characterized by strong translational ordering in the second shell, a feature that is absent in ordinary simple fluids. To illustrate this point we plot in Fig. 1b the same probability distribution for a hard-sphere fluid at the largest supercooling before the onset of spontaneous crystallization (pressure βPσ 3 =17, above the melting pressure βPσ 3 ≃ 11.5 (ref. 29 )). The distribution is monotonically decreasing, showing no translational ordering (for comparison, the distribution of the fcc crystal phase is plotted). The shape of P ( d f–s ) of water at low temperatures ( Fig. 1a ) has a maximum at finite d f–s and then increases again at d f–s =0 due to shell interpenetration, that is, non-hydrogen-bonded oxygen atoms that are closer to the central oxygen atom than the hydrogen-bonded neighbours. In our model, the structuring of the fluid at low temperatures is interpreted as an increase in locally favoured structures. 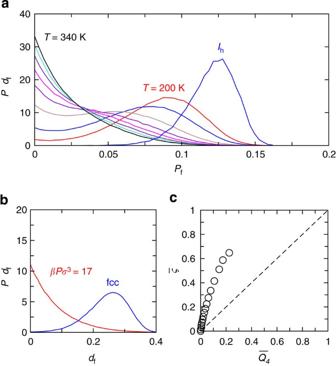Figure 1: Structuring of the second shell in supercooled water. (a) Probability distribution of the distance between the first and second shell,df–s, defined as the difference between the radial distances of the fifth and fourth nearest oxygen neighbours to the central oxygen atom. The state points go fromT=340 to 200 K (with intervals of 20 K), at ambient pressure. Also depicted is the probability distribution for hexagonal ice (Ih) at ambient pressure andT=200 K. The figure shows that on cooling water molecules progressively acquire more structure, with the formation of a finite separation between the first two shells, anticipating the full order found in the solid phase (Ih). (b) Probability distributions of the distance between the first and second shell,df–s, for a hard spheres fluid at reduced pressureβPσ3=17 (whereσis the diameter of the spheres) and for an fcc crystal.df–sis defined as the difference between the radial distances of the 13th and 12th nearest neighbours. Differently from the case of water, simple fluids do not show evidence of translational ordering of the second shell on supercooling. (c) Evolution of the average translational order parameterand of the average orientational orderfor water at ambient pressure and temperatures ranging fromT=350 to 200 K. Both order parameters are normalized as to be 0 in the high temperature state (T=350 K) and 1 in the solidIhphase atT=200 K. The dashed straight line represents the relation of. Figure 1: Structuring of the second shell in supercooled water. ( a ) Probability distribution of the distance between the first and second shell, d f–s , defined as the difference between the radial distances of the fifth and fourth nearest oxygen neighbours to the central oxygen atom. The state points go from T =340 to 200 K (with intervals of 20 K), at ambient pressure. Also depicted is the probability distribution for hexagonal ice ( I h ) at ambient pressure and T =200 K. The figure shows that on cooling water molecules progressively acquire more structure, with the formation of a finite separation between the first two shells, anticipating the full order found in the solid phase ( I h ). ( b ) Probability distributions of the distance between the first and second shell, d f–s , for a hard spheres fluid at reduced pressure βP σ 3 =17 (where σ is the diameter of the spheres) and for an fcc crystal. d f–s is defined as the difference between the radial distances of the 13th and 12th nearest neighbours. Differently from the case of water, simple fluids do not show evidence of translational ordering of the second shell on supercooling. ( c ) Evolution of the average translational order parameter and of the average orientational order for water at ambient pressure and temperatures ranging from T =350 to 200 K. Both order parameters are normalized as to be 0 in the high temperature state ( T =350 K) and 1 in the solid I h phase at T =200 K. The dashed straight line represents the relation of . Full size image Locally favoured structures correspond to local structures with low energies E , high specific volumes υ and low degeneracy g . In the following, we denote these structures as the S state. In contrast, thermally excited states are characterized by a high degree of disorder and degeneracy, low specific volumes and high energies. We label these structures as the ρ state. In formulas, υ ρ < υ S , E S < E ρ and g S << g ρ . To identify the S state, we introduce a new order parameter ζ , which measures local translational order in the second shell of neighbours, hinted from the behaviour of P ( d f–s ) shown in Fig. 1a . The importance of the second shell structure was notably pointed out by Soper and Ricci [48] . Translational order is a measure of the relative spacing between neighbouring particles, and it is one of the fundamental symmetries broken at the liquid-to-solid transition [29] . Locally, a molecule is in a state of high translational order if the radial distribution of its neighbours is ordered. A liquid, by definition, cannot have full translational order, but it might display translational order on shorter scales. Water molecules, even at high temperatures, display a high level of tetrahedral symmetry, indicatig that a high degree of translational order is always present up to the first shell of nearest neighbours. In this sense, tetrahedral order itself is not enough to describe water’s anomalies. To determine locally favoured states, we focus instead on ‘translational order of second nearest neighbours’. The operational definition goes as follows (a schematic representation is given in Fig. 2a ). For water molecule i (labelled 0 in Fig. 2a ), we order its neighbours according to the radial distance d ji of the oxygen atoms; the order parameter ζ ( i ) is then defined as the difference between the distance d j ′ i of the first neighbour not hydrogen bonded to i (with label 5 in the figure) and the distance dj ′′ i of the last neighbour hydrogen bonded to i (labelled 4 ). Two oxygen atoms are considered hydrogen bonded if the distance between donor (D) and acceptor (A) is within 0.35 nm, and the angle H-D-A is less than 30° (ref. 47 ). Our order parameter might apparently look similar to another microscopic structural order parameter introduced by Poole and his coworkers [37] , that is, the radial distribution function of the fifth oxygen atom, but a crucial difference comes from whether hydrogen bonding is considered in addition to the distance measure or not (see Supplementary Fig. 1 and Supplementary Note 1 ). As we will show, the S state having high translational symmetry, is characterized by large values of ζ , with a clear separation between first and second shell (for example, when the fifth molecule is in position 5 in Fig. 2a ). However, these structures should not be confused with local crystalline structures, as they generally lack orientational order, that is, the neighbours in the second shell are not oriented according to the crystal directions (with well-defined eclipsed and staggered configurations) owing to their embedding in water’s disordered network. The average value of ζ in both the cubic and hexagonal ice structures at T =200 K and P =1 bar is ζ =0.122, which is higher (as we will show) than the average for the S states. In the ρ state, the second shell is collapsed, with a distribution of ζ values roughly centred around ζ =0 (in Fig. 2a this state is obtained, for example, when the fifth neighbour is in position 5′ ) and comprising many configurations with negative values of ζ , resulting from the penetration of the first shell from an oxygen atom belonging to a distinct tetrahedra. 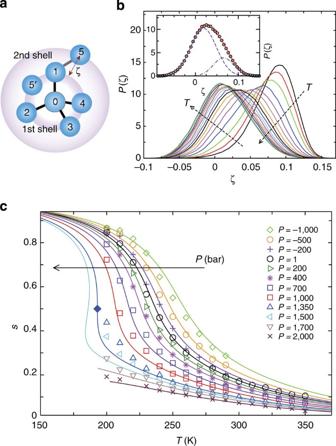Figure 2:T,Pdependence of the structural order parameter. (a) Schematic representation of the local environment around a water molecule (labelled0), showing the position of the hydrogen-bonded molecules that form the first shell (with labels from1to4). Also depicted is the closest non-hydrogen-bonded molecule for two different states: theSstate, when the fifth neighbour is in position5, so that there is a clear separation between first and second shell, with the order parameterζrepresenting the distance between them; theρstate, with the fifth neighbour in position5′, so that the second shell is collapsed onto the first one. (b) Distribution function of the order parameterζat ambient pressure (P=1 bar) and at different temperatures. The temperatures range fromT=200 to 350 K in steps of 10 K (the arrows indicate increasing temperatures). The inset shows the distribution function atT=280 K obtained from the simulations (circle symbols), and the decomposition in two Gaussian populations: theρpopulation in dashed line, theSpopulation in dashed-dotted line and the sum of both populations in the continuous (red) line. (c) Values of the fraction of theSstate (s) as a function of temperature for all simulated pressures. The symbols are the values obtained by the decomposition of the order parameter distribution,P(ζ), at the corresponding state point. Continuous lines are fits according to the two-state model, with the following parameters defined in the text:a1=−2.90 × 102,a2=−9.00 × 101,a11=−6.32 × 102,a12=−1.23 × 102anda22=−1.86 × 101. The full diamond shows the location of the critical point,Tc=1.93,Pc=1,350 (ref.46). Figure 2: T , P dependence of the structural order parameter. ( a ) Schematic representation of the local environment around a water molecule (labelled 0 ), showing the position of the hydrogen-bonded molecules that form the first shell (with labels from 1 to 4 ). Also depicted is the closest non-hydrogen-bonded molecule for two different states: the S state, when the fifth neighbour is in position 5 , so that there is a clear separation between first and second shell, with the order parameter ζ representing the distance between them; the ρ state, with the fifth neighbour in position 5′ , so that the second shell is collapsed onto the first one. ( b ) Distribution function of the order parameter ζ at ambient pressure ( P =1 bar) and at different temperatures. The temperatures range from T =200 to 350 K in steps of 10 K (the arrows indicate increasing temperatures). The inset shows the distribution function at T =280 K obtained from the simulations (circle symbols), and the decomposition in two Gaussian populations: the ρ population in dashed line, the S population in dashed-dotted line and the sum of both populations in the continuous (red) line. ( c ) Values of the fraction of the S state ( s ) as a function of temperature for all simulated pressures. The symbols are the values obtained by the decomposition of the order parameter distribution, P ( ζ ), at the corresponding state point. Continuous lines are fits according to the two-state model, with the following parameters defined in the text: a 1 =−2.90 × 10 2 , a 2 =−9.00 × 10 1 , a 11 =−6.32 × 10 2 , a 12 =−1.23 × 10 2 and a 22 =−1.86 × 10 1 . The full diamond shows the location of the critical point, T c =1.93, P c =1,350 (ref. 46 ). Full size image For hard spheres, the structural ordering in the liquid state is characterized by orientational order rather than translational order [25] , [26] , [28] , [29] , [49] . Unlike the case of hard spheres, in the supercooled state water develops translational order much faster than orientational order. This is shown in Fig. 1c where the average normalized translational order, , and orientational order, , of the second shell are plotted for several state points at ambient pressure. Q 4 is a standard measure of orientational order, and its mathematical definition is given in the Methods section and ref. 29 . The order parameters and are normalized to be 0 at high temperature ( T =350 K) and 1 in the crystal phase at T =200 K. The difference between a hard-sphere liquid and water comes from the fact that water has a very high orientational and translational ordering in the first shell because of hydrogen bonding. The spatial arrangement of this tetrahedral units is the key to characterize the water structure and best captured by the translational ordering in the second shell, which takes into account hydrogen-bonding patterns. Two-state model of water At ordinary thermodynamic conditions, the two states ( S and ρ ) are mixed and the free energy ( G ) of the mixture takes the form of a regular solution, that is, the simplest non-ideal model of liquid mixture [23] . where s is the fraction of the S state, G α ( α = ρ , S ) is the free energy of the pure component, Δ G = G S − G ρ and J is the coupling between the two states, that is, the source of non-ideality. Unlike ordinary regular solutions, the fraction s is not fixed externally, but by the equilibrium of the conversion reaction between the two states, ρ S , obtained by equating their chemical potentials ( μ S = μ ρ ) If J >0 the mixing is endothermic, and the model displays a critical point at k B T c = J /2, below which the system undergoes a liquid–liquid demixing transition. A two-state model for the thermodynamic anomalies requires a definition of Δ G . Since this term is Δ G =0 at the LLCP, we use as a second-order Taylor expansion around the location of the LLCP [46] . When fitting the values of s obtained from simulations with equation (2), we thus have five independent fitting parameters (see Methods section for their definition). Two-state model of microscopic configurations Figure 2b shows the probability distribution of the order parameter ζ at ambient pressure ( P =1 bar) and for different temperatures, ranging from T =200 to 350 K. The distribution shows a remarkable non-monotonic change (of both height and width) with temperature. This behaviour can be rationalized by decomposing the distribution function in two Gaussian populations, each varying monotonically with temperature (see Methods for the details). An example of this decomposition is shown in the inset of Fig. 2b for the distribution function at T =280 K, which is close to the state point of density maximum. The ρ population (dashed line in the inset of Fig. 2b ) is centred in proximity of ζ =0, meaning that there is a large fraction of configurations in which the first shell (defined as the hydrogen-bonded molecules to the central molecule) is being penetrated by oxygen atoms belonging to different tetrahedral units. The S population is instead characterized by high values of ζ , having a well-formed second shell. The fitting procedure produces a reliable decomposition for state points having s <70% ( s is the fraction of the S state in the model of equation (1)) where the fitting parameters are well behaved. This covers the whole region of the phase diagram accessible to experiments. Howeveer, for deeply supercooled states at low pressures (below T ≈230 K at ambient pressure), the fraction of the ρ state becomes small, and the estimation of s from unconstrained fits becomes more difficult (see Methods). Nonetheless, as we will show later, the predictions of the model for the deeply supercooled states are still in good agreement with simulations. T , P -dependence of the structural order parameter From the decomposition we can extract the fraction of the S state in the liquid, that is, the parameter s in the two-state model of equation (1). The values of s extracted from all simulated state points are shown in Fig. 2c . For any pressure, the fraction of the S state increases monotonically by lowering the temperature, and the increase is steeper at lower pressures. At low temperatures, we can see a big jump in the values of s between P =1,000 bar and P =1,350 bar. This could signal the close presence of a LLCP. In fact, previous studies of TIP4P/2005 water (and with the same system size) have determined its location at T c =193 K and P c =1,350 bar (ref. 46 ), although the exact location of the critical point and even its existence are still ambiguous [13] , [50] . Next, we fit the two-state model of equation (2) to our simulation results (see Methods for the details of the fitting). The results of the fit are shown as continuous lines in Fig. 2c , demonstrating that the two-state model provides a very good representation of the microscopic structure-based results obtained from simulations (represented by symbols in the same figure). Note that the agreement holds to very high temperatures, and for all pressures, suggesting a strong microscopic basis for the relevance of our order parameter. This is in stark contrast to previous attempts to obtain a two-state description of water from microscopic information [37] , [44] , [45] , where the agreement was restricted to the deeply supercooled region. We note that most of previous models have unphysical saturations of the value of s at high temperature around 0.5 or even higher, unlike our model where s <<1 at high temperatures (see also refs 25 , 26 for a review). It is also worth mentioning that the only region of significant discrepancy is limited around the critical point, which is due not only to the higher uncertainty in accessing s around the critical region, but possibly also to critical fluctuations that are not incorporated in the present mean-field two-state model (but which is possible with a crossover theory [36] ) or an imprecise location of the critical point [13] , [50] . Two-state description of water anomalies We will now check whether the two-state picture extracted so far can account for water’s anomalies. From the free energy of equation (1), it is possible to derive the anomalous contribution to density, which takes the form ρ = N / V with V = V ρ + s Δ V , where V ρ is the volume of N molecules of the pure ρ state and Δ V is the average volume difference between S state and ρ state. The term Δ V is fixed by the two-state model, and fitting the anomalies requires modelling the term V ρ for the density dependence of a non-anomalous liquid, which we do with a quadratic function in ρ , , where only the term b 0 is pressure dependent (so that fitting a new isobar requires a single fitting parameter). For more details on the T – P dependence of Δ V and V ρ , see Methods. 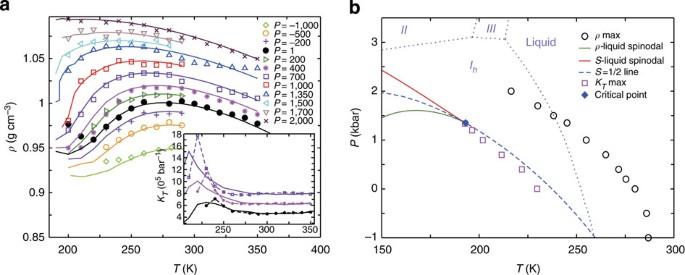Figure 3: Thermodynamic and phase behaviour of water. (a) Temperature dependence of density for several pressures. Continuous lines are simulation results, while symbols are obtained from the two-state model. The inset shows the compressibility forP=1,400,700 bar: dashed lines are simulation results, while symbols are two-state model predictions. The curves in the inset are traslated on theyaxis to improve readability. (b) Phase diagram of the two-state model. The Widom line (dashed line) is by definition the line wheres=1/2. The compressibility maximum (squares) from simulations lies close to the Widom line, eventually converging at the critical point (full diamond). Below the critical point the two components undergo macroscopic phase separation. The spinodals of the transition are denoted with full lines: green for theρliquid and red for theSliquid. Circles show the locus of density maximum, which continuously increases as water is stretched, in agreement with experiments at extreme negative pressures62. Dotted lines show the location of the coexisting lines between the liquid and different forms of ice taken from ref.63. Figure 3a shows density isobars measured in simulations (continuous lines) that are compared with the results from the two-state model (symbols). We can see that the two-state model correctly represents the intensity and location of the density anomaly for all studied pressures (with the anomaly disappearing at high pressures). The agreement is more remarkable in the relevant region of the anomalies, while it is approximate at very low temperatures (for which we know the estimation of s being subject to higher uncertainty). For example, the model predicts a density minimum at around 220 K at ambient pressure (full circles in Fig. 3a ), which is found instead at 200 K in simulations. The inset shows the isothermal compressibility κ T for pressures P =1,400,700 bar. As in the main figure, continuous lines are direct simulation results, showing the rapid increase at low temperatures, while symbols are predictions from the model (see Methods). Isothermal compressibility anomalies are much harder to describe accurately, both because compressibility is a second derivative of the model’s free energy, G (see Methods), thus suffering bigger uncertainty, and also because its anomaly is located at very low temperatures, where it is more difficult to get reliable estimation of the fraction s . Nonetheless, as shown in the inset of Fig. 3a , the model predicts within 10 K the location of the compressibility maximum, and also its increased intensity at higher pressures (eventually diverging at the critical point). Figure 3: Thermodynamic and phase behaviour of water. ( a ) Temperature dependence of density for several pressures. Continuous lines are simulation results, while symbols are obtained from the two-state model. The inset shows the compressibility for P =1,400,700 bar: dashed lines are simulation results, while symbols are two-state model predictions. The curves in the inset are traslated on the y axis to improve readability. ( b ) Phase diagram of the two-state model. The Widom line (dashed line) is by definition the line where s =1/2. The compressibility maximum (squares) from simulations lies close to the Widom line, eventually converging at the critical point (full diamond). Below the critical point the two components undergo macroscopic phase separation. The spinodals of the transition are denoted with full lines: green for the ρ liquid and red for the S liquid. Circles show the locus of density maximum, which continuously increases as water is stretched, in agreement with experiments at extreme negative pressures [62] . Dotted lines show the location of the coexisting lines between the liquid and different forms of ice taken from ref. 63 . Full size image Phase behaviour of TIP4P/2005 water We summarize the phase behaviour of the two-state model in the phase diagram of Fig. 3b . The Widom line of the model, where s =1/2, lies close to the compressibility maximum line obtained from simulations (open squares), with the two lines converging at the critical point. Here we note that the location of the Widom line is determined by the condition Δ G ( T , P )=0, that is, the two-state feature without cooperativity (see equation (2)). This indicates that the isothermal compressibility anomalies in this temperature range are not due to critical phenomena associated with LLCP, but due to the sigmoidal change in s characteristic of the two-state model (Schottky-type anomaly) [23] , [24] , [25] , [26] . Also shown in the phase diagram are the spinodals (or stability limits) of the S liquid and the ρ liquid, which in the LLCP scenario are usually called the low-density liquid and the high-density liquid, respectively. Phase behaviour of TIP5P water To show that the previous results are not unique to the TIP4P/2005 potential, in this section we consider the TIP5P potential, a five-point, rigid, non-polarizable water model [51] . 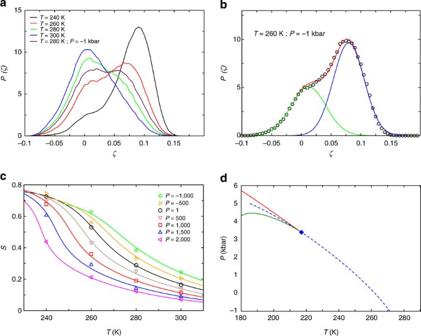Figure 4: Two-state analysis for the TIP5P model of water. (a) Probability distribution function for the order parameterζfor state points atP=1 bar, and forP=−1 kbar atT=260 K. (b) Distribution function atT=206 K andP=−1 kbar obtained from the simulations (circle symbols), and the decomposition in two Gaussian populations: theρpopulation in green, theSpopulation in blue and the sum of both populations in the red line. (c) Values of the fraction of theSstate (s) as a function of temperature for all simulated pressures. The symbols are the values obtained by the decomposition of the order parameter distribution,P(ζ), at the corresponding state point. Continuous lines are fits according to the two-state model, with the following parameters defined in the text:a1=−5.84 × 102,a2=−1.52 × 102,a11=−2.59 × 103,a12=−1.02 × 103anda22=−1.30 × 102. (d) Phase diagram of TIP5P from the two-state model. The Widom line is the dashed line wheres=1/2. The full diamond shows the location of the critical point,Tc=217 K,Pc=3,400 bar (ref.52). The spinodals of the transition are denoted with full lines: green for theρliquid and red for theSliquid. Figure 4a plots the probability distribution function P ( ζ ) for several state points. When compared with the ones for the TIP4P/2005 potential ( Fig. 2b ), the distribution functions of the TIP5P potential show a more clear bimodality, with a component centred around ζ ∼ 0 (the ρ state) and the other centred at a finite value of ζ (the S state). An example of the decomposition of P ( ζ ) in two Gaussian populations is shown in Fig. 4b . The fraction s of the S state for several state points is shown in Fig. 4c , together with the two-state model fits (continuous lines). Figure 4d plots the predicted phase diagram with the Widom line (dashed line) and the two spinodals (continuous lines). For the critical point ( T c =217 K and P c =3,400 bar), we use the estimate obtained in ref. 52 . Figure 4: Two-state analysis for the TIP5P model of water. ( a ) Probability distribution function for the order parameter ζ for state points at P =1 bar, and for P =−1 kbar at T =260 K. ( b ) Distribution function at T =206 K and P =−1 kbar obtained from the simulations (circle symbols), and the decomposition in two Gaussian populations: the ρ population in green, the S population in blue and the sum of both populations in the red line. ( c ) Values of the fraction of the S state ( s ) as a function of temperature for all simulated pressures. The symbols are the values obtained by the decomposition of the order parameter distribution, P ( ζ ), at the corresponding state point. Continuous lines are fits according to the two-state model, with the following parameters defined in the text: a 1 =−5.84 × 10 2 , a 2 =−1.52 × 10 2 , a 11 =−2.59 × 10 3 , a 12 =−1.02 × 10 3 and a 22 =−1.30 × 10 2 . ( d ) Phase diagram of TIP5P from the two-state model. The Widom line is the dashed line where s =1/2. The full diamond shows the location of the critical point, T c =217 K, P c =3,400 bar (ref. 52 ). The spinodals of the transition are denoted with full lines: green for the ρ liquid and red for the S liquid. Full size image Pair correlation functions The microscopic approach described in the previous sections requires the knowledge of the instantaneous positions of both oxygen and hydrogen atoms in the system, thus being suitable only for computational studies. Here we show that, with minor approximations, it is possible to obtain the fraction of the S state not only from the distribution of ζ but also from experimentally measurable quantities, which can probe the degree of translational order. The definition of ζ involves the difference between the distance of the first non-hydrogen-bonded oxygen and the last hydrogen-bonded oxygen. The hydrogen bond interaction is a limited range interaction and breaks when the oxygen atoms involved in the bond are too far apart. We call this cutoff distance r H-bond . In our simulation study, we have set this distance at r H-bond =0.35 nm (ref. 47 ). This means that if we look at two oxygen atoms whose distance is about r H-bond , these atoms (with high probability) do not share a hydrogen bond. At the same time we know that in the S state the first non-hydrogen-bonded atom has a vanishing small probability to be at distances close to the first neighbours’ shell ( ζ =0). It follows that the contribution to the radial distribution function at distance r H-bond comes predominantly from the ρ state. To clarify this point, we consider the radial distribution functions of oxygen atoms, g ( r ), plotted in Fig. 5a . Continuous lines show the radial distribution function for different state points along the Widom line (where by definition s =1/2): the distributions are all very close to each other, with an isosbestic point approximately at r H-bond =0.35 nm. The reason for the isosbestic point is that, as noted above, the value of the radial distribution function at r H-bond is proportional to the fraction of the ρ state, and this is constant at the Widom line. Coincidentally, the value of the radial distribution function at r H-bond is approximately g ( r H-bond )=0.5, suggesting a direct proportionality between the fraction of the ρ state and g ( r H-bond ). This is confirmed by plotting the radial distribution functions of state points with a low fraction of the ρ state ( P =−1,000 bar, T =200 K, dotted dashed line) and a high fraction of ρ state ( P =2,000 bar, T =350 K, dashed line), where the value of g ( r H-bond ) is found to be close to 0 and 1, respectively. We thus write the following relation between the height of g ( r ) and s (the fraction of the S state): s ≅ 1− g ( r H-bond ). 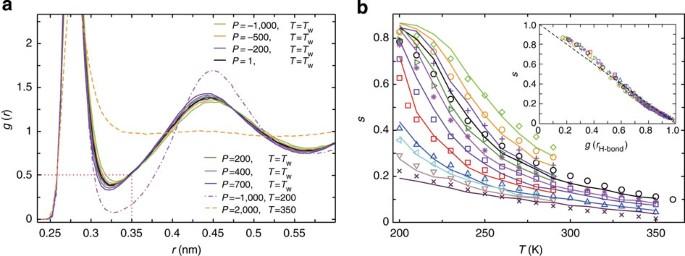Figure 5: Estimation ofsfrom the radial distribution function of oxygen atomsg(r). (a) Radial distribution functiong(r) for state points along the Widom lineTW(P) (continuous lines). The functions were obtained by linear interpolation of radial distribution functions of the closest simulated state points. Also plotted are the radial distribution functions of two-state points with respectively a high fraction of theSstate (P=−1,000 bar,T=200 K, dotted dashed line) and a high fraction ofρstate (P=2,000 bar,T=350 K, dashed line). The dotted lines denote the isosbestic point close torH-bond=0.35 nm. (b) Comparison between the values ofs: symbols represent values obtained from the relations≅1−g(rH-bond), while lines are the values obtained from the distribution function of the order parameterζ(the lines in this figure represent the same data as the symbols inFig. 2c). The inset shows the comparison between the value ofsobtained from the distribution function of the order parameterζand the value ofg(rH-bond) at the same state points. Figure 5b compares the results of this relation with the results obtained by fitting the distribution function of the order parameter ζ . In the inset, these two values are plotted for all state points considered in this work, showing that indeed the relation s =1− g ( r H-bond ) holds to a good approximation. The main panel in Fig. 5b shows the temperature dependence of these two values, showing again the good agreement between the two calculation methods. Note that the relation s =1− g ( r H-bond ) seems to hold better for s <0.5, which is the same range that the experiments are able to access. This opens up a possibility to estimate the structural order parameter, that is, the degree of translational order in the second shell, from scattering experiments. Figure 5: Estimation of s from the radial distribution function of oxygen atoms g ( r ). ( a ) Radial distribution function g ( r ) for state points along the Widom line T W ( P ) (continuous lines). The functions were obtained by linear interpolation of radial distribution functions of the closest simulated state points. Also plotted are the radial distribution functions of two-state points with respectively a high fraction of the S state ( P =−1,000 bar, T =200 K, dotted dashed line) and a high fraction of ρ state ( P =2,000 bar, T =350 K, dashed line). The dotted lines denote the isosbestic point close to r H-bond =0.35 nm. ( b ) Comparison between the values of s : symbols represent values obtained from the relation s ≅ 1− g ( r H-bond ), while lines are the values obtained from the distribution function of the order parameter ζ (the lines in this figure represent the same data as the symbols in Fig. 2c ). The inset shows the comparison between the value of s obtained from the distribution function of the order parameter ζ and the value of g ( r H-bond ) at the same state points. Full size image Microscopic structural features of locally favoured structures We now investigate the microscopic features of locally favoured states. We have shown that the S state can be identified with configurations having a high degree of translational order, indicating that second nearest neighbours are at approximately the same distance from the central oxygen atom. We now discuss the orientational order of second nearest neighbours. Crystalline configurations are characterized by full orientational order, with second nearest neighbours occupying the characteristic eclipsed and staggered orientations present in the stable ice I c and I h polymorphs (see Fig. 6a ). To investigate the structure of the S state, we consider only oxygen atoms for which our order parameter ζ is in the range ζ ε[0.075, 0.1125], where the S population peaks (see Fig. 2 ). We also exclude from the analysis particles that are identified as belonging to small crystals that spontaneously form and dissolve in a supercooled melt. To identify crystalline particles, we use standard order parameters based on Steinhardt rotational invariants [53] , [54] . For each of the oxygen atoms previously defined, we determine the optimal rotation that minimizes the following root mean square deviation , where r i ( i =1 ∼ 4) are the unitary vectors joining the central oxygen atom ( r 0 ) with its four nearest neighbours, and v i ( i =1 ∼ 4) are the directions of a reference tetrahedron, given by v 0 =(0, 0, 0), , , and v 4 =(0, 0, 1). The same rotation is applied to second nearest neighbours, defined as all oxygen atoms whose distance from any of the first nearest neighbours is within 1.2 times the average oxygen–oxygen distance. We then compute the probability distribution for the position of second nearest neighbours in spherical coordinates, according to the usual transformations: , θ =cos −1 ( z / r ) and φ =tan −1 ( y / x ), where z is the axis connecting the central oxygen atom with the closest vertex v i of the regular tetrahedron. A schematic representation of the coordinate system is shown in Fig. 6a . 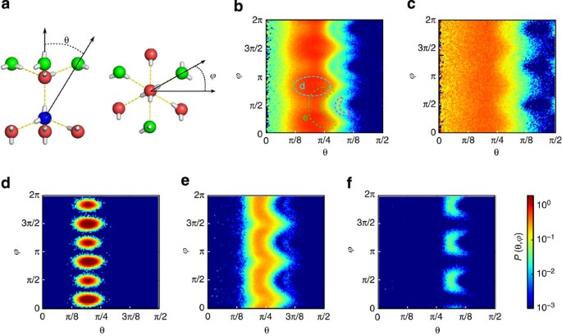Figure 6: Structure of theSstate. (a) Polar maps of the relative position of second nearest neighbours (green oxygen atoms) of a given molecule (blue oxygen atom), with its first nearest neighbours (red oxygen atoms) oriented so to minimize the mean square distance from a regular tetrahedron (see text for details). (b) Liquid state atT=200 K andP=1 bar. Only particles that are not identified as crystalline, and withζε[0.075, 0.1125] are plotted. The dashed labelled lines are guides to the structures into which theSstate can be decomposed, and which are plotted in the corresponding panels. (c) The same as in panelb, but for the state pointT=280 K andP=1 bar. (d) Hexagonal ice (Ih) atT=200 K andP=1 bar. (e) Liquid state atT=200 K andP=1 bar, where only particles belonging to five-membered rings are plotted. (f) Liquid state atT=200 K andP=1 bar, where only particles belonging to four-membered rings are plotted. The colour bar represents the probability density for panelsb,c,eandf, which are all computed from the same set of configurations. Figure 6: Structure of the S state. ( a ) Polar maps of the relative position of second nearest neighbours (green oxygen atoms) of a given molecule (blue oxygen atom), with its first nearest neighbours (red oxygen atoms) oriented so to minimize the mean square distance from a regular tetrahedron (see text for details). ( b ) Liquid state at T =200 K and P =1 bar. Only particles that are not identified as crystalline, and with ζ ε[0.075, 0.1125] are plotted. The dashed labelled lines are guides to the structures into which the S state can be decomposed, and which are plotted in the corresponding panels. ( c ) The same as in panel b , but for the state point T =280 K and P =1 bar. ( d ) Hexagonal ice ( I h ) at T =200 K and P =1 bar. ( e ) Liquid state at T =200 K and P =1 bar, where only particles belonging to five-membered rings are plotted. ( f ) Liquid state at T =200 K and P =1 bar, where only particles belonging to four-membered rings are plotted. The colour bar represents the probability density for panels b , c , e and f , which are all computed from the same set of configurations. Full size image Typical results for equilibrium configurations are shown in Fig. 6 (see also Supplementary Fig. 2 and Supplementary Note 2 ). To aid the understanding of these plots, we first report in Fig. 6d the results for the hexagonal ice crystal. The six well-defined peaks correspond to the possible positions of second nearest neighbours in the crystal, showing full orientational order: larger peaks correspond to staggered configurations, whereas smaller peaks correspond to eclipsed configurations. In Fig. 6b , we plot the results for the S state of liquid water at T =200 K and P =1 bar. We first notice that the full orientational order found in the crystal is lost in the S state. Nevertheless, one can still identify structural patterns that characterize the S state, and that are marked by the dashed lines in Fig. 6b . The first pattern denoted as region ‘d’ surrounded by the white dashed line corresponds to staggered arrangements of molecules, providing strong evidence that the S state is a precursor of crystallization, that is, it is along the microscopic pathway that water undergoes when transforming from liquid to solid. The second prominent structural pattern found in the S state is denoted as region ‘e’ surrounded by the green dashed line in Fig. 6b and it is not found in stable ice crystals. This pattern is centred around eclipsed configurations but it is characterized by fluctuations that are distinct from the one found in the hexagonal crystal. While second nearest neighbours in crystalline configurations are involved in loops of six hydrogen-bonded oxygen atoms, the pattern denoted as region ‘e’ is instead due to five-membered rings. This is shown in Fig. 6e where only oxygen atoms belonging to five-membered rings are plotted, displaying the same pattern found in the S state. Although in much less quantity, there are also four-membered rings as indicated by the pattern ‘f’ in Fig. 6b , as confirmed in Fig. 6f , where only oxygen atoms belonging to four-membered rings are plotted. Roles of locally favoured structures in ice crystallization Pentagonal rings, loops of five water molecules bonded to each other through hydrogen bonding act as the source of frustration against crystallization [25] , [26] , [55] , [56] . To crystallize, the S structure needs first to break a hydrogen bond and then orient its neighbours along the crystal’s directions. The S state is energetically stable with respect to the disordered ρ state (since each pentagon ring adds one hydrogen bond to the structure) but pays a high entropic cost owing to the missing degrees of freedom when closing a ring. Pentagon rings could then be responsible for the high degree of supercooling reachable with water, stabilizing the S state and frustrating the direct crystallization transition to hexagonal and cubic ices. Region ‘f’ surrounded by the pink dashed line represent four-member rings, which are plotted in Fig. 6f and are present in far less extent than five-member rings. Thus, the S state is characterized by mixed structural signatures, one of which is consistent with the crystal structure and the other is not. We investigate the statistics of five-membered rings in Fig. 7 . The first panel shows some snapshots of pentagonal rings for configurations having, respectively, one, two, three and four five-membered rings. For each S structure, the maximum number of pentagonal rings is six. In Fig. 7b , we show how the fraction of pentagonal rings in the S structures changes with temperature, for different values of the pressure. The number of five-membered rings increases with decreasing temperature and pressure. A decrease in temperature increases the population of the S state, so favouring crystallization, but this is partly counterbalanced by an increase in five-membered rings. The importance of the presence of five-membered rings in the S state for crystallization of water will be discussed in more detail elsewhere. 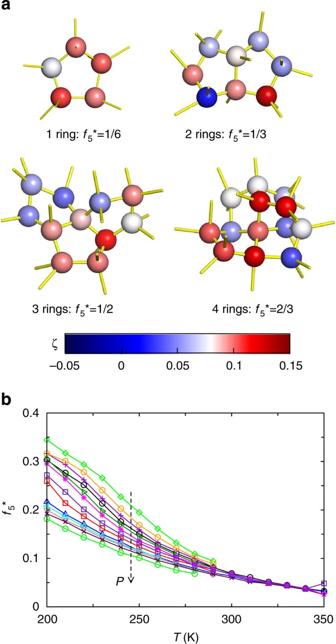Figure 7: Pentagonal rings. (a) Snapshots of water configurations with, respectively, one, two, three and four five-membered rings. Oxygen atoms are coloured according to the value of the translational order parameterζ. (b) Fraction of pentagonal rings in theSstructures, as a function ofTfor all pressures considered in the letter. The order of increasing pressure is indicated by the dashed arrow. Figure 7: Pentagonal rings. ( a ) Snapshots of water configurations with, respectively, one, two, three and four five-membered rings. Oxygen atoms are coloured according to the value of the translational order parameter ζ . ( b ) Fraction of pentagonal rings in the S structures, as a function of T for all pressures considered in the letter. The order of increasing pressure is indicated by the dashed arrow. Full size image To conclude, we have provided a microscopic description of water’s anomalies based on locally favoured states defined as structures with local translational order. Microscopically, these states reflect the underlying crystallization behaviour of water. Owing to its strong directional bonding, the crystallization pathway of water can be approximated in two steps: in the first step, water develops translational order, which is reflected in the population of S states; in the second step, it develops orientational order where the hydrogen bonds in the shell of second nearest neighbours acquire the staggered and eclipsed configurations, which characterize the hexagonal and cubic forms of ice. The S state is a locally favoured state (energetically stabilized) with a high abundance of pentagonal rings, loops of five particles bonded to each other through hydrogen bonding. Five-membered rings increase with lowering the temperature and thus act as a source of frustration against crystallization into hexagonal and cubic ices [25] , [26] , [55] , [56] . The model that results from this framework is compatible with water’s anomalies over a wide range of temperatures and pressures. The viability of a two-state model from microscopic configurations was tested for both TIP4P/2005 and TIP5P potentials. In the context of the LLCP scenario, the low-density liquid and high-density liquid states would be, respectively, the S -dominant and ρ -dominant states below the critical point. In fact, the order parameter ζ includes the local configurations responsible for water’s two-length scales average interaction [3] . It shows also strong analogies with the concept that network interpenetration can sustain one or multiple LLCPs [57] . On the other hand, we note that, within the two-state model, the presence of a critical point associated with demixing is not a necessary condition for the existence of thermodynamic anomalies, and the anomalies survive even if the mixture lacks a critical point, ( J =0 in equation (1)) [23] . Such a possibility, i.e. the lack of a critical point, has recently been suggested for TIP4P/2005 water [13] , [50] . We stress that the parameters of the model were obtained only from microscopic information, and then its predictions were compared with the anomalies of water. It would be possible also to use the model in a phenomenological way, by fitting the anomalies to improve the model parameters, for example, improving the estimates in the deeply supercooled region (obtaining better estimates for the density minimum and the isothermal compressibility maximum). In this work we have avoided such an approach to show that a two-state description of the phase behaviour of water is possible based solely on microscopic information. Once this is confirmed, precision fitting of the anomalies can provide additional insights [24] , [36] . Successful two-state descriptions of related water models, like the ST2 potential [38] and the mW potential [41] also suggest the viability of this approach. For this reason, we have also provided an approximate scheme to extract the model’s parameters from experimentally accessible measurements. Knowledge of the oxygen–oxygen radial distribution function is in fact accessible with both neutron and X-ray scattering methods (see, for example, ref. 58 ). Performing these measurements over a wide range of temperatures and pressures could provide important information, such as the nature of the non-idealities of the mixture (for example, whether they have an energetic or entropic origin [36] ). Here it may be worth noting the roles of locally favoured structures in crystallization. We show that locally favoured structures in water not only have translational order in the second shell, but also contain five-membered rings of hydrogen-bonded molecules, indicating a mixed character of their roles in crystallization: the former helps crystallization, whereas the latter causes frustration against crystallization into hexagonal and cubic ices. This frustration effect may be related with the rather large degree of supercooling of water before homogenous crystal nucleation takes place. Finally, our approach could be useful not only in studies of pure water but also in water mixtures, where a liquid–liquid transition of the water component has been observed [19] , or in water–salt solutions, where the effect of salt on the structure of water is similar to the effect of pressure [59] , [60] . We can further speculate that the two-state model based on the translational order of the second shell may be relevant also to other tetrahedral liquids (Si, Ge, silica, germania) [25] , [26] , [61] , which play a crucial role in materials science. Molecular dynamics simulations Molecular dynamics simulations were run using the Gromacs (v.4.5) molecular dynamics simulation package. The isothermal-isobaric NPT ensemble was sampled through a Nosé–Hoover thermostat and an isotropic Parrinello–Rahman barostat. Lennard–Jones interactions have a cutoff at 0.95 nm, and cutoff corrections are applied to both energy and pressure. Electrostatic interactions are calculated through Ewald summations, with the real part being truncated at 0.95 nm, and the reciprocal part evaluated using the particle mesh method. The systems consist of 512 molecules of water, and the total simulation time varied from 200 ns for the high temperature simulations up to 1 μs for the lowest temperatures. We use both the TIP4P/2005 (ref. 46 ) and the TIP5P (ref. 51 ) force fields for water. Hydrogen bonds are located through geometric constraints on the relative positions of the donor (D), acceptor (A) and hydrogen (H) atom. Two oxygen atoms are considered hydrogen bonded if their distance is within 0.35 nm, and the angle H-D-A is less than 30° (ref. 47 ). Analysis of the distribution function P ( ζ ) The distribution function P ( ζ ) is decomposed in two Gaussian populations. To distinguish unambiguously two Gaussian populations with large overlap, we take into account the fact that one of the two populations (corresponding to the S state) should be characterized by fully formed translational order up to second shell, so its distribution should be vanishingly small for ζ →0 + . This means that the S state is characterized by good translational order on both first and second shells. Imposing this constraint on the fitting, we are able to decompose the distribution in two populations for a large region of the phase diagram. The fitting function satisfying the above constraint is given by where m ρ , σ ρ , m S , σ S are the fitting parameters. Both m ρ and m S are monotonically decreasing with temperature, showing that states become more and more structured at low temperatures, while σ ρ and σ S are increasing with temperature, as expected by the increase of thermal fluctuations. The function is obtained by decomposing P ( ζ ) into two Gaussian P ( ζ )=(1− s ) P ρ ( ζ )+ sP S ( ζ ), under the constraint P S (0)=0, which is rationalized by the fact that for the S state the fifth water molecule closest to the central one must be hydrogen bonded to a water molecule in the first shell. The fitting performs well for state points characterized by s ≲ 0.7 (so, throughout the experimentally accessible region), but at very low temperatures and pressures the fraction of the ρ state becomes very small, increasing the uncertainty of the fit. One possible way to overcome these difficulties is by noting that the ρ fluid should behave like a fluid without anomalies, and thus its parameters ( m ρ and σ ρ ) should be well-behaved functions of P and T . We then choose to estimate the value of m ρ with a quadratic extrapolation from the values obtained at state points with s ≲ 0.7. This procedure degrades the accuracy of the model only at the lowest temperatures and for small pressures (as can be seen in the estimates for the isothermal compressibility maximum and the minimum in density in Fig. 3a ), but the agreement with simulations is still satisfactory. Note instead that the TIP5P model is characterized by a more clear bimodality ( Fig. 4a ), and the decomposition can be obtained directly from equation (3) for all state points considered. Fitting of the T – P dependence The two-state model predictions are based on the free energy expression given by equation (1). To fully specify the model, an expression for the free energy difference between the two bulk states, Δ G , has to be provided. In our model this difference is expressed as a second-order expansion around the known location of the LLCP: where and . We employ T c =193 K and P c =1,350 bar, which are reported for the same system [46] . This also fixes the value of J =2 k B T c . The coefficients of the expansion a αβ are given in the caption of Fig. 2 . The resulting free energy allows the calculation of the anomalous term of any thermodynamic property A , that is, the difference between the value of A in the mixture and its value in a pure state (the background), A ρ or A S . We define the anomalous term, Δ A , with the following expression: A = A ρ + s Δ A . For example, the expressions for the density and compressibility anomalies are found, respectively, with first- and second-order derivatives of the free energy with respect to pressure The calculation of the absolute value of the thermodynamic properties requires a reasonable assumption on the T – P dependence of the background part, which is usually written as a low-order polynomial. For example, . We stress that the success of a two-state model depends on the ability to determine the location and intensity of the anomalies that do not depend on the knowledge of the background terms. Orientational order Q 4 A (2 l +1) dimensional complex vector ( q l ) is defined for each particle i as , where we set l =4, and m is an integer that runs from m =−1 to m =1. The functions Y lm are the spherical harmonics and is the normalized vector from the oxygen of molecule i to one of the molecule j . The sum goes over the first N b ( i )=16 neighbours of molecule i . This choice accounts for the first two coordination shells of tetrahedral crystals. We then introduce a spatial coarse-graining step . Finally, Q 4 ( i ) is defined as the following rotational invariant . How to cite this article: Russo, J. and Tanaka, H. Understanding water’s anomalies with locally favoured structures. Nat. Commun. 5:3556 doi: 10.1038/ncomms4556 (2014).